Wide-band quantum interface for visible-to-telecommunication wavelength conversion Although near-infrared photons in telecommunication bands are required for long-distance quantum communication, various quantum information tasks have been performed by using visible photons for the past two decades. Recently, such visible photons from diverse media including atomic quantum memories have also been studied. Optical frequency down-conversion from visible to telecommunication bands while keeping the quantum states is thus required for bridging such wavelength gaps. Here we report demonstration of a quantum interface of frequency down-conversion from visible to telecommunication bands by using a nonlinear crystal, which has a potential to work over wide bandwidths, leading to a high-speed interface of frequency conversion. We achieved the conversion of a picosecond visible photon at 780 nm to a 1,522-nm photon, and observed that the conversion process retained entanglement between the down-converted photon and another photon. Photons have an important role for transmitting a quantum state among distantly located physical systems, such as atoms, ions and solid-state systems [1] , [2] , [3] , [4] , which are used as memories and/or processors of quantum communication [5] , [6] and information processing [7] . So far, experimental demonstrations aiming at such tasks have been actively done with photons in visible wavelengths [8] , [9] . However, when we look at long-distance quantum communication [10] , a near-infrared wavelength within telecommunication bands is vital for efficient optical fibre communications. This optical frequency mismatch can be filled by frequency conversion of a photon while preserving its quantum state [11] . A pioneer work of such a quantum interface for the optical frequency conversion has been done by using a second-order nonlinearity in a periodically-poled LiNbO 3 (PPLN) crystal [12] , in which a photon of a telecom wavelength was up-converted to a visible one. Such a frequency up-conversion was also actively studied for efficient detection of photons in telecommunication bands [13] . On the other hand, quantum interfaces for frequency down-conversion from visible to telecommunication bands have recently been demonstrated by using a third-order nonlinearity of a dense atomic cloud [14] , [15] , which uses two pump lights MHz-detuned from resonant frequencies of the atom. In these demonstrations, choice of the target wavelength is severely limited to the vicinity of the resonant frequency of the atom. Such a restriction on frequency selections can be relaxed by using a bulk nonlinear crystal. So far, aiming at such a versatile quantum interface, demonstrations of difference-frequency generation (DFG) in nonlinear optical crystals with a strong pump and a weak coherent light seed have been performed [16] , [17] . In this paper, we present the first demonstration of DFG-based frequency down-conversion of non-classical light by a nonlinear optical crystal from a visible wavelength at 780 nm to a telecommunication wavelength at 1,522 nm. Using a waveguided PPLN crystal with a wide acceptable bandwidth as the second-order nonlinear optical material, we have observed sub-Poissonian photon statistics of the light at 1,522 nm after the frequency down-conversion of a picosecond single-photon pulse at 780 nm. Then, we have demonstrated the frequency down-conversion of one half of a 780-nm-entangled photon pair, and observed the entanglement between the down-converted photon at 1,522 nm and the other half at 780 nm. Basic concept The quantum theory of frequency conversion of single-mode pulsed light using a second-order nonlinear optical interaction is as follows. When the pump light at angular frequency ω p is sufficiently strong, the quantum dynamics of a signal mode at angular frequency ω s and a converted mode at angular frequency ω c satisfying ω c = ω s − ω p is described by the following Hamiltonian: where â s and â c are annihilation operators of the signal mode and the converted mode, respectively. A coupling constant ξ =| ξ | e i φ of the nonlinear optical medium is proportional to the complex amplitude of the classical pump light, where φ is the phase of the pump light. Using the Heisenberg representation with , annihilation operators â s,out and â c,out of the signal and converted modes coming out from the nonlinear medium are written as and where τ is the travelling time of the pulses through the nonlinear medium. The process of the frequency conversion described in equations (2) and (3) can be regarded as a beamsplitter in the frequency degree of freedom with the transmittance of cos 2 (| ξ | τ ). A condition | ξ | τ = π /2 for the complete conversion is achieved by adjusting the amplitude of the pump light and the length of the nonlinear medium. Estimation of the conversion efficiency with a classical light As a preliminary experiment, we performed the frequency down-conversion of a classical light in a coherent state. 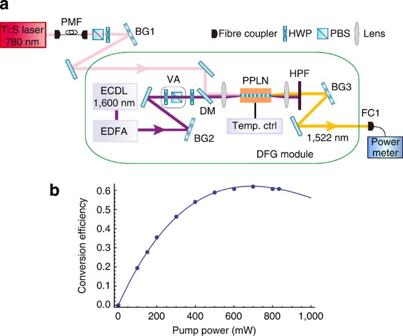Figure 1: Frequency down-conversion of coherent light pulse. (a) Experimental setup. The signal light from the mode-locked Ti:sapphire (Ti:S) laser at 780 nm and the pump beam from the ECDL at 1,600 nm are combined at the dichroic mirror (DM). Then they are coupled into the PPLN for the frequency down-conversion to the 1,522-nm wavelength. The light at 1,522 nm is extracted using the high-pass filter (HPF) and the BG3 with a 1-nm bandwidth, and coupled to the single-mode fibre. EDFA, Erbium-doped fibre amplifier; VA, variable attenuator; Temp. ctrl, temperature control. (b) The conversion efficiency depending on the power of the pump light coupled to the PPLN. The maximum conversion efficiency ≈0.62 was obtained at 700-mW pump power. A solid curve is fitted using a functionexpected from equation (2), wherePpumpis the pump power. ParametersAandBare estimated as 0.62 and 3.6 mW−1, respectively. Our experimental setup is shown in Figure 1a . We use a mode-locked Ti:sapphire laser as a signal light source. The centre wavelength is 780 nm, the pulse width is 1.2 ps and the repetition rate is 82 MHz. After passing through a polarization-maintaining fibre (PMF), the signal beam is set to vertical (V) polarization by a polarization beamsplitter (PBS) and a half-wave plate (HWP). The signal beam is diffracted by a Bragg grating (BG1), which narrows the bandwidth to 0.2 nm. A seed laser beam from an external cavity diode laser (ECDL) at 1,600 nm with a linewidth of Δ f ≡150 kHz is amplified by an Erbium-doped fibre amplifier, and then it is used as a pump light for the DFG. We use BG2 with the bandwidth of 1 nm for suppressing unnecessary frequency components of the pump light. The power of the pump light is adjusted by a variable attenuator composed of a HWP and a PBS. The signal and pump lights are set to V polarization and combined at a dichroic mirror, and then focused on the PPLN crystal. Details of the PPLN are described in Methods section. Figure 1: Frequency down-conversion of coherent light pulse. ( a ) Experimental setup. The signal light from the mode-locked Ti:sapphire (Ti:S) laser at 780 nm and the pump beam from the ECDL at 1,600 nm are combined at the dichroic mirror (DM). Then they are coupled into the PPLN for the frequency down-conversion to the 1,522-nm wavelength. The light at 1,522 nm is extracted using the high-pass filter (HPF) and the BG3 with a 1-nm bandwidth, and coupled to the single-mode fibre. EDFA, Erbium-doped fibre amplifier; VA, variable attenuator; Temp. ctrl, temperature control. ( b ) The conversion efficiency depending on the power of the pump light coupled to the PPLN. The maximum conversion efficiency ≈0.62 was obtained at 700-mW pump power. A solid curve is fitted using a function expected from equation (2), where P pump is the pump power. Parameters A and B are estimated as 0.62 and 3.6 mW −1 , respectively. Full size image After passing through the PPLN waveguide, the strong pump light is diminished by a high-pass filter and the converted light at 1,522 nm is extracted by BG3 with a bandwidth of 1 nm. Finally, the beam is coupled into a single-mode fibre by a fibre coupler (FC1) and connected to a power meter. This setup gave us the overall conversion efficiency from the 780-nm photon coupled in the PPLN to the 1,522-nm photon coupled to the fibre, which took its maximum 0.39 at 700-mW pump power. The transmittance of the optical components from the end of the PPLN to the power meter was estimated to be ≈0.62, which is calculated from the diffraction efficiency 0.88 of BG3 and the coupling efficiency 0.71 to FC1. Using the transmittance, the photon conversion efficiency of the PPLN was estimated to be 0.62 at 700 mW, and its pump power dependence is shown in Figure 1b . The conversion efficiency will be improved when the linewidth of the signal light becomes much narrower than the acceptable linewidth of the PPLN waveguide. When we used a 780-nm CW light from an ECDL with a 3-MHz linewidth, we observed the maximum conversion efficiency of 0.71. Preservation of sub-Poissonian photon statistics The preservation of the photon statistics of the signal light after the frequency conversion is the first step towards the demonstration of our quantum interface [18] , [19] . Non-classical behaviour of the photon statistics of the pulsed light appears in the second-order intensity correlation function between the n th neighbour pulses defined by where Î ( t ) is an intensity operator at time t , T is the time interval of the pulses and the integrations are over a range of the single-pulse duration. The product of the operators is in normal order and time order [20] . While is always satisfied in the classical wave theory, the quantization of light allows the possibility that is smaller than 1, with the smallest value for an ideal single-photon pulse. 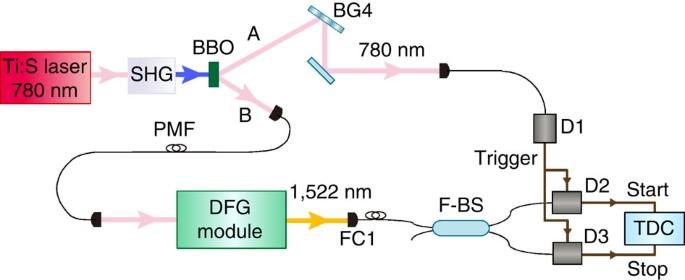Figure 2: Frequency down-conversion of heralded single photons at 780 nm. The light pulse from the Ti:sapphire (Ti:S) laser is frequency doubled to the wavelength of 390 nm by second harmonic generation (SHG), and then pumps a type-I phase-matched 1.5 mm-thick β-barium borate (BBO) crystal to prepare a photon pair A and B at 780 nm by spontaneous parametric down-conversion. The photon in mode A is detected by a silicon avalanche photodiode detector D1 connected to a single-mode fibre for the preparation of the heralded single photon in mode B. We observe the second-order intensity correlation functionof the light converted to 1,522 nm using the Hanbury–Brown and Twiss setup (Methods). F-BS, fibre-optic beamsplitter. The experimental setup for frequency down-conversion of a single photon at 780 nm followed by correlation measurement on the converted light is shown in Figure 2 . A photon pair A and B are generated by spontaneous parametric down-conversion at a β -barium borate crystal, and the presence of a single photon in mode B is heralded by detection of a photon in mode A by a photon detector D1. The spectral filtering of the photon in mode A is performed by BG4 with a bandwidth of 0.2 nm. The wavelength of the heralded single photon is converted to 1,522 nm by the DFG module described in Figure 1a . The converted pulse is then coupled to FC1 and its intensity correlation is measured with two InGaAs/InP avalanche photodiodes D2 and D3 (see Methods). Figure 2: Frequency down-conversion of heralded single photons at 780 nm. The light pulse from the Ti:sapphire (Ti:S) laser is frequency doubled to the wavelength of 390 nm by second harmonic generation (SHG), and then pumps a type-I phase-matched 1.5 mm-thick β-barium borate (BBO) crystal to prepare a photon pair A and B at 780 nm by spontaneous parametric down-conversion. The photon in mode A is detected by a silicon avalanche photodiode detector D1 connected to a single-mode fibre for the preparation of the heralded single photon in mode B. We observe the second-order intensity correlation function of the light converted to 1,522 nm using the Hanbury–Brown and Twiss setup (Methods). F-BS, fibre-optic beamsplitter. Full size image The measured of the light converted from the heralded single photon at 780 nm was 0.17±0.04, which is much smaller than 1, and indicates sub-Poissonian photon statistics of the converted light. This result clearly shows that the non-classical property of the light survived after the frequency down-conversion. The non-zero value of is mainly caused by optical noises from the PPLN. They are linearly increasing with the pump power when the signal light is turned off, which may suggest that they are caused by Raman scattering [21] . Conversion of entangled photons Finally, we performed the frequency down-conversion of one halves of polarization-entangled photon pairs at 780 nm. 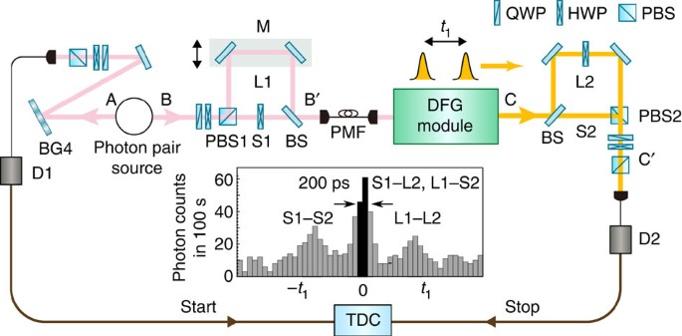Figure 3: Frequency down-conversion of one halves of polarization-entangled photon pairs. At the photon pair source, the light pulse from the Ti:sapphire (Ti:S) laser is frequency doubled by second harmonic generation, and pumps a pair of β-barium borate crystals to prepare the entangled photon pair |φ+›ABthrough spontaneous parametric down-conversion22. The frequency down-conversion of photon B is performed after encoding a polarization qubit into a time-bin qubit using an unbalanced MZI, then decoding it back to the polarization qubit after frequency down-conversion. The histogram shows the number of coincidence events with various delay between the detectors D1 and D2, which were recorded by the TDC. The measurement bases of photons in modes A and C′ are set as +45° polarization. The central peak shows the events where the photon has passed through S1–L2 or L1–S2, and the two peaks separated from the central peak byt1correspond to the cases where the photon has passed through S1–S2 or L1–L2. We accept the events in 200-ps time window around the central peak as the successful events. The experimental setup is shown in Figure 3 . A photon pair source prepares a polarization-entangled photon pair A and B described as . The spectral filtering of photon A is performed by BG4. Photon B goes to an unbalanced Mach–Zehnder interferometer (MZI). At the MZI, PBS1 separates H and V polarization into a short path (S1) and a long path (L1), respectively. After horizontal (H) polarization is flipped to V polarization by a HWP inserted into S1, modes S1 and L1 are mixed by a BS. This transforms the polarization qubit in mode B to a time-bin qubit in mode B′, and the initial two-photon state | φ + › AB becomes a polarization and time-bin-entangled state Figure 3: Frequency down-conversion of one halves of polarization-entangled photon pairs. At the photon pair source, the light pulse from the Ti:sapphire (Ti:S) laser is frequency doubled by second harmonic generation, and pumps a pair of β-barium borate crystals to prepare the entangled photon pair | φ + › AB through spontaneous parametric down-conversion [22] . The frequency down-conversion of photon B is performed after encoding a polarization qubit into a time-bin qubit using an unbalanced MZI, then decoding it back to the polarization qubit after frequency down-conversion. The histogram shows the number of coincidence events with various delay between the detectors D1 and D2, which were recorded by the TDC. The measurement bases of photons in modes A and C′ are set as +45° polarization. The central peak shows the events where the photon has passed through S1–L2 or L1–S2, and the two peaks separated from the central peak by t 1 correspond to the cases where the photon has passed through S1–S2 or L1–L2. We accept the events in 200-ps time window around the central peak as the successful events. Full size image where |S1› and |L1› represent the states of the V-polarized photons passing through S1 and L1, respectively. After passing through a PMF, the photon in mode B′ goes to the DFG module. The light down-converted by the DFG process inherits the phase − φ of the pump light as described in equation (2). Then, through the frequency down-conversion, the former and the latter term in equation (5) receive phase shifts − φ ( t ) and − φ ( t + t 1 ) from the pump light, respectively. In our experiment, as t 1 is about 1 ns and Δ f is 150 kHz, the coherence time 1/(2 π Δ f )≈1 μ s of the pump light is much longer than t 1 , which ensures that φ ( t )=− φ ( t + t 1 ) is satisfied. As a result, we should obtain the state | ψ › AC for the 780-nm photon and the 1,522-nm photon in mode C. The down-converted photon in mode C is fed to the second unbalanced MZI. A BS in the MZI divides the converted photon into a short path (S2) and a long path (L2). A HWP inserted in L2 flips the polarization from V to H. Two modes S2 and L2 are recombined by PBS2. This transforms the degree of freedom from time-bin to polarization. After the MZI, the photon in mode C′ goes to detector D2, which is gated by trigger counts from D1. The path lengths S1–L2 and L1–S2 are adjusted by the mirrors M on a motorized and piezo-driven stage. When we post-select the events where the photon has passed through S1–L2 or L1–S2, we should obtain the polarization-entangled state | φ + › AC′ for the two photons in modes A and C′. In our experiment, we accept such events in 200-ps time window shown in the histogram in the inset of Figure 3 . We first performed quantum state tomography of 780-nm photon pairs in modes A and B from the photon pair source. The required polarization correlations have been measured by rotating a quarter-wave plate and a HWP in mode A, and a quarter-wave plate and a HWP before PBS1 in mode B [23] . The PMF before the DFG module was connected to a silicon avalanche photodiode. We observed the two-photon state with a detection rate of 492 Hz. 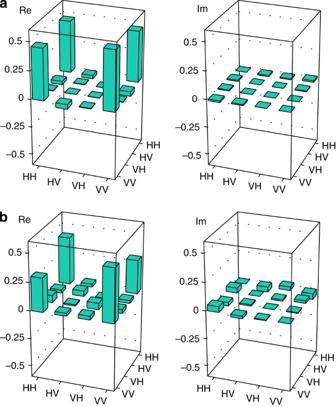Figure 4: The reconstructed density matrices. (a) The initial entangled photon pairρABprepared by the photon pair source. (b) The two-photon stateρAC′between the 780-nm photon in mode A and the 1,522-nm photon in mode C′. The overall detection rate of each photon pairρABandρAC′is 492 and 2.4 Hz, respectively. The reconstructed density operator ρ AB is shown in Figure 4a . The iterative maximum likelihood method was used for the reconstruction of ρ AB [24] , [25] . The observed fidelity of ρ AB to | φ + › AB was 0.95±0.01, which implies that the photon pair source prepared a highly entangled 780-nm photon pair. Next, we performed quantum state tomography of the photon in mode A and the converted photon in mode C′. Here, a detection rate of the two photons was 2.4 Hz. The reconstructed density operator ρ AC′ of the state is shown in Figure 4b . We calculated the fidelity and entanglement of formation [26] from reconstructed ρ AC′ as 0.75±0.06 and 0.36±0.13, respectively. The observed value of the fidelity is greater than , which implies that the entangled state ρ AC′ can violate the Clauser–Horne–Shimony–Holt inequality. We note that when we subtract background noises whose rate is about 0.8 Hz from the observed coincidence counts, the fidelity of the output state becomes 0.95, which shows that the degradation is mainly caused by the optical noises from the PPLN. Figure 4: The reconstructed density matrices. ( a ) The initial entangled photon pair ρ AB prepared by the photon pair source. ( b ) The two-photon state ρ AC′ between the 780-nm photon in mode A and the 1,522-nm photon in mode C′. The overall detection rate of each photon pair ρ AB and ρ AC′ is 492 and 2.4 Hz, respectively. Full size image In the current experiment, the two-photon detection rate was 1.6 Hz, resulting from the subtraction of the background noises 0.8 Hz. As the quantum efficiency of the silicon avalanche photodiode is about 0.6 at 780 nm and that of the InGaAs/InP avalanche photodiode is about 0.25 at 1,522 nm, the overall conversion efficiency of photons just before the photon detector is estimated to be 1.6 Hz×0.6/(492 Hz×0.25)≈0.008. This value is much smaller than 0.39 observed for the laser light. This inefficiency is caused by the complicated experimental setup for the frequency down-conversion of the entangled photon pair. The conversion efficiency from time-bin to polarization qubit is below 0.5. Post-selection efficiency for extracting the events only within 200-ps time-bin was about 0.5. We put the filtering grating only in mode A, which leads to a broader spectrum of the converted telecom single photon than that of the classical light. This results in the conversion efficiency inside the PPLN to be about 0.14, due to the limited acceptance linewidth of the phase matching. Moreover, several optics were added in the setup, and an additional fibre was inserted after the FC to add a time delay for the gate operation of the detector D2. The transmittance of the optical components is expected to drop from 0.62 to about 0.2. We consider that the above inefficiencies degrade the net conversion efficiency for the entangled photon pairs. In our experiment, the degradation of the fidelity was mainly caused by the optical noise. We believe that it is caused by anti-Stokes Raman scattering of the CW pump light. Here, we discuss three practical solutions to reduce it. The first solution is to use a measurement system with a faster time resolution. In our current experiment, the converted photon passed through the spectral filter BG3 whose bandwidth is 1 nm, which corresponds to about 4-ps time duration. On the other hand, due to the poor timing resolution of our detectors and time-to-digital converter (TDC), the data were accumulated during 200 ps, which increased the background counts caused by the optical noises. Therefore, instruments with faster time resolution allow us to reduce the noise counts. To the best of our knowledge, superconducting detectors have achieved a timing resolution <20 ps, which will improve the signal-to-noise ratio by a factor of 10. This will give a high fidelity around 0.9. The second solution is the use of a photon with narrower spectrum and a narrower filtering of a converted light for avoiding the photons from the Raman scattering with the broad spectrum. In the case of a converted light with a linewidth 0.1 times that in the current experiment, we may use a filter with one-tenth bandwidth to reduce the noise photons by a factor of 10, resulting in a high fidelity around 0.9. Finally, cooling the PPLN crystal will be a more direct way to reduce the number of photons from the anti-Stokes Raman scattering. Cooling down the PPLN to around 130 K, we expect to reduce the noise photons to one-tenth. In conclusion, we have demonstrated the frequency down-conversion of non-classical light at 780 nm to a telecommunication wavelength of 1,522 nm by using the DFG process in the PPLN waveguide. Our quantum interface has down-converted the frequency of one half of the visible entangled photon pair to the telecommunication wavelength while preserving entanglement. The DFG process with the quasi-phase-matching techniques allows us to convert a wide range of visible wavelengths to telecommunication ones with a wide acceptable bandwidth. We believe that such a quantum interface will be useful for long-distance quantum communication based on various visible photon emitters. Details of the PPLN waveguide The PPLN waveguide in our experiments consists of Zn-doped lithium niobate as the waveguide core and lithium tantalite as the cladding layer [27] . The waveguide is a ridged type with 8-μm wide, and its length is 20 mm. The periodically-poled structure has an 18-μm period designed for the type-0 quasi-phase matching. The best conversion efficiency was obtained at the temperature of 50°C. The acceptable phase-matching bandwidth for the 780-nm signal light of the 20-mm long crystal is calculated to be about 0.3 nm. Measurement of intensity correlation g 0 (2). As shown in Figure 2 , the second-order intensity correlation g 0 (2) of the down-converted pulse is measured by using a Hanbury–Brown and Twiss setup [28] , [29] , which consists of a fibre-optic beamsplitter and photon detectors D2 and D3 gated by trigger signals from D1. To measure the temporal difference between the detections at D2 and D3 with high resolution, signals from D2 and D3 are input to a TDC as a start and a stop signal of the clock, respectively. By recording the trigger counts N trig from D1, the start counts N start from D2, the stop counts N stop from D3 and coincidence counts N coinc within 1 ns from the TDC, we determine g 0 (2) by How to cite this article : Ikuta, R. et al . Wide-band quantum interface for visible-to-telecommunication wavelength conversion. Nat. Commun. 2:537 doi: 10.1038/ncomms1544 (2011).